Convergent evolution of plant pattern recognition receptors sensing cysteine-rich patterns from three microbial kingdoms The Arabidopsis thaliana Receptor-Like Protein RLP30 contributes to immunity against the fungal pathogen Sclerotinia sclerotiorum . Here we identify the RLP30-ligand as a small cysteine-rich protein (SCP) that occurs in many fungi and oomycetes and is also recognized by the Nicotiana benthamiana RLP RE02. However, RLP30 and RE02 share little sequence similarity and respond to different parts of the native/folded protein. Moreover, some Brassicaceae other than Arabidopsis also respond to a linear SCP peptide instead of the folded protein, suggesting that SCP is an eminent immune target that led to the convergent evolution of distinct immune receptors in plants. Surprisingly, RLP30 shows a second ligand specificity for a SCP-nonhomologous protein secreted by bacterial Pseudomonads. RLP30 expression in N. tabacum results in quantitatively lower susceptibility to bacterial, fungal and oomycete pathogens, thus demonstrating that detection of immunogenic patterns by Arabidopsis RLP30 is involved in defense against pathogens from three microbial kingdoms. To survive attacks by harmful microbes, plants have evolved a multifaceted innate immune system [1] , [2] , [3] . Pattern recognition receptors (PRRs) that perceive pathogen/microbe-associated molecular patterns (PAMPs/MAMPs) at the plasma membrane play an important role in this system to initiate active defense responses [3] , [4] , [5] , [6] . Many PRRs contain leucine-rich repeat (LRR) ectodomains. Based on the presence or absence of a cytoplasmic kinase domain, these LRR-PRRs can be classified as receptor kinases (LRR-RKs) or receptor-like proteins (LRR-RPs), respectively [3] , [4] , [5] , [6] . Immunity-related LRR-RPs form constitutive complexes with the common adapter kinase SOBIR1 (SUPPRESSOR OF BRASSINOSTEROID INSENSITIVE 1 (BRI1)-ASSOCIATED KINASE (BAK1)-INTERACTING RECEPTOR KINASE 1), thus forming bi-molecular equivalents of LRR-RKs [4] , [7] . Upon binding their specific PAMP ligands, the LRR-RP/SOBIR1 complexes, much like the LRR-RKs, recruit co-receptors of the SERK (SOMATIC EMBRYOGENESIS RECEPTOR KINASE) family such as BAK1 for activation of intracellular immune signaling and induction of defense responses [4] , [8] . Over the past decades, a number of PAMP/PRR pairs have been identified [3] , [4] , [6] , [9] and most of these PAMPs occur only in a single kingdom of microorganisms. However, there are notable exceptions including the XEG1-type glucanohydrolases and the VmE02-type cysteine-rich proteins which are conserved in many plant-pathogenic fungi and oomycetes, or NLPs (NEP1-(NECROSIS AND ETHYLENE-INDUCING PEPTIDE 1)-LIKE PROTEINS) which are present in bacterial, fungal and oomycete species [10] , [11] , [12] , [13] . Perception of PAMPs is often restricted to closely related species, reflecting a vast diversity in the repertoires of PRRs between plant families. Restriction to closely related species holds for LRR-RP-type PRRs of Arabidopsis , including RLP23, RLP32 and RLP42, which sense nlp20, proteobacterial TRANSLATION INITIATION FACTOR 1 (IF1) and fungal polygalacturonases (PGs), respectively [4] , [14] , [15] . These LRR-RPs have no obvious homologs in species outside the Brassicaceae family. Likewise, LRR-RPs identified in solanaceous plants such as tomato, including EIX2 (ETHLYENE-INDUCING XYLANASE RECEPTOR 2) and the Cf proteins detecting effectors from Cladosporium fulvum have no counterparts in species of other plant families [4] . Intriguingly, detection of only a few PAMPs, notably bacterial flagellin by FLAGELLIN-SENSING 2 (FLS2) and fungal chitin by CHITIN-ELICITOR RECEPTOR KINASE 1 (CERK1), occurs in a broad range of plant species [16] , [17] . The Arabidopsis Receptor-Like Protein 30 (RLP30) mediates basal resistance to the fungus Sclerotinia sclerotiorum but the identity of the proteinaceous PAMP detected by RLP30 remained open [18] . Here, we report the identification of this factor as a SMALL CYSTEINE-RICH PROTEIN (SCP) closely related to VmE02 from Valsa mali [12] . Apart from sensing SCPs from different fungi and oomycetes, RLP30 can recognize an SCP-unrelated pattern from Pseudomonas bacteria and confers increased resistance to Nicotiana tabacum plants. We further reveal distinct immune-sensing mechanisms for SCPs in Brassicaceae and Solanaceae species. Our findings unveil an unanticipated complex relationship between PRRs and PAMPs where a single PRR recognizes PAMPs from microorganisms of three kingdoms and where a single PAMP is detected by phylogenetically distinct PRRs from different plant species. SCP Ss is the immunogenic pattern secreted by S. sclerotiorum The Arabidopsis RLP30 detects a proteinaceous elicitor secreted by S. sclerotiorum , originally termed SCFE1 [18] . To identify the immunogenic pattern in the supernatants of fungal cultures, we used an extended fractionation protocol and monitored fractions for RLP30-dependent induction of the plant stress hormone ethylene (Supplementary Fig. 1a, b ). 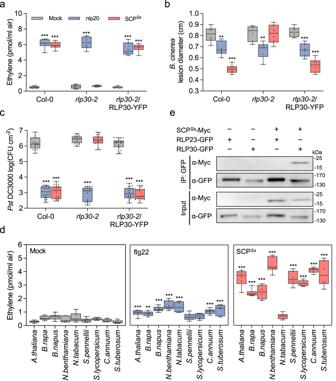Fig. 1: SCPSsis immunogenic and binds to RLP30. aEthylene accumulation inArabidopsisCol-0 wild-type plants,rlp30-2mutants, or anrlp30-2line complemented with ap35S::RLP30-YFPconstruct 4 h after treatment with water (mock), 1 μM nlp20, or 1 µMP. pastoris-expressed SCPSs.bB. cinereainfected area as determined by lesion diameter on day 2 after 24 h-treatment of Col-0 wild-type plants,rlp30-2mutants or therlp30-2/RLP30-YFPcomplementation line with water (mock), 1 µM nlp20, or 1 µM SCPSs.cBacterial growth in plants pre-treated with water (mock), 1 μM nlp20, or 1 μM SCPSs24 h before infiltration ofPstDC3000. Bacteria (colony forming units, CFU) were quantified in extracts of leaves 3 days after inoculation.dEthylene accumulation in plants of the Brassicaceae and Solanaceae family 4 h after treatment with water (mock), 1 μM flg22, or 1 µM SCPSs.eLigand-binding assay inN. benthamianatransiently co-expressing SCPSs-myc and either RLP30-GFP or RLP23-GFP. Leaf protein extracts (Input) were used for co-immunoprecipitation with GFP-trap beads (IP:GFP) and immunoblotting with tag-specific antibodies. Fora–d, data points are indicated as dots (n= 6 fora,b,d;n= 20 for c) and plotted as box plots (center line, median; bounds of box, the first and third quartiles; whiskers, 1.5 times the interquartile range; error bar, minima and maxima). Statistically significant differences from mock treatments in the respective plants are indicated (two-sided Student’sttest, **P≤ 0.01, ***P≤ 0.001). Source data are provided as a Source data file. All assays were performed at least three times with similar results. Mass spectrometric analysis of the trypsin fragments obtained with the ethylene-inducing fractions revealed the presence of a small cysteine-rich protein (Sscle06g048920; SMALL CYSTEINE-RICH PROTEIN FROM S. SCLEROTIORUM , SCP Ss ) of 147 amino acids containing eight cysteine residues but no known protein domains (Supplementary Table 1 and Supplementary Fig. 1c ). To confirm SCP Ss as the ligand of RLP30, the SCP Ss protein was heterologously expressed in N. benthamiana or Pichia pastoris (Supplementary Fig. 1d, e ), with C-terminal GFP or His tags, respectively. Both forms were found to induce ethylene production in Arabidopsis Col-0 wild-type plants but not in the rlp30-2 mutant (Fig. 1a and Supplementary Fig. 1f ), ruling out that contaminations occurring during the purification procedure or SCP Ss -copurifying proteins are responsible for the RLP30-dependent defense response. His-tagged SCP Ss , affinity purified via His-Trap columns, triggered ethylene production in Col-0 plants at nanomolar concentrations with a half-maximal induction (EC 50 ) at ~26 nM (Supplementary Fig. 2a ). In contrast to rlp30-2 mutants, Col-0 wild-type plants and rlp30-2 mutants complemented with RLP30 responded to the SCP Ss preparations with typical PAMP responses such as induction of reactive oxygen species (ROS), activation of mitogen-activated protein kinases (MAPK), and a generally induced state of resistance, supported by significantly reduced colonization by the fungus Botrytis cinerea or the bacterial pathogen Pseudomonas syringae pv. tomato ( Pst ) DC3000 (Fig. 1b, c and Supplementary Fig. 2b, c ). Unlike most other known patterns recognized by RPs, SCP Ss did not only elicit ethylene production in Arabidopsis and related Brassica species, but also in solanaceous plants such as N. benthamiana , tomato, pepper, and potato (Fig. 1d ). Fig. 1: SCP Ss is immunogenic and binds to RLP30. a Ethylene accumulation in Arabidopsis Col-0 wild-type plants, rlp30-2 mutants, or an rlp30-2 line complemented with a p35S::RLP30-YFP construct 4 h after treatment with water (mock), 1 μM nlp20, or 1 µM P. pastoris -expressed SCP Ss . b B. cinerea infected area as determined by lesion diameter on day 2 after 24 h-treatment of Col-0 wild-type plants, rlp30-2 mutants or the rlp30-2/RLP30-YFP complementation line with water (mock), 1 µM nlp20, or 1 µM SCP Ss . c Bacterial growth in plants pre-treated with water (mock), 1 μM nlp20, or 1 μM SCP Ss 24 h before infiltration of Pst DC3000. Bacteria (colony forming units, CFU) were quantified in extracts of leaves 3 days after inoculation. d Ethylene accumulation in plants of the Brassicaceae and Solanaceae family 4 h after treatment with water (mock), 1 μM flg22, or 1 µM SCP Ss . e Ligand-binding assay in N. benthamiana transiently co-expressing SCP Ss -myc and either RLP30-GFP or RLP23-GFP. Leaf protein extracts (Input) were used for co-immunoprecipitation with GFP-trap beads (IP:GFP) and immunoblotting with tag-specific antibodies. For a – d , data points are indicated as dots ( n = 6 for a , b , d ; n = 20 for c) and plotted as box plots (center line, median; bounds of box, the first and third quartiles; whiskers, 1.5 times the interquartile range; error bar, minima and maxima). Statistically significant differences from mock treatments in the respective plants are indicated (two-sided Student’s t test, ** P ≤ 0.01, *** P ≤ 0.001). Source data are provided as a Source data file. All assays were performed at least three times with similar results. Full size image To assess whether SCP Ss can be found in complex with RLP30, co-immunoprecipitation assays were performed with extracts from N. benthamiana leaves that were transiently co-transformed with myc-tagged SCP Ss and with either GFP-tagged RLP30 or the GFP-tagged nlp20 receptor RLP23 [19] as control. SCP Ss -myc co-precipitated specifically with RLP30 but not with the structurally related RLP23 (Fig. 1e ). Several Arabidopsis accessions that were found to exhibit no response to S. sclerotiorum extracts carry single nucleotide polymorphisms in their RLP30 genes leading to single amino acid changes [18] . In an extended screen with 77 accessions, we identified further accessions that did not respond to SCP Ss and that carried point mutations in RLP30 (Supplementary Figs. 3a and 4 ). We tested the altered RLP30 versions occurring in these insensitive accessions in a co-precipitation assay for binding of SCP Ss . While most receptor versions, except RLP30 from Sq-1 and Lerik1-3, were expressed in N. benthamiana , none of them precipitated SCP Ss (Supplementary Fig. 3b ). Thus, the single amino acid substitutions in different parts of the LRR and island domains, which are specific to SCP Ss -responsive RLP30 variants [18] , such as L307R in Mt-0, R433G in Lov-1 and Lov-5, R433L in ICE111, N561Y in Bak-2, G563V in Br-0, and F760 in Gu-0 (Supplementary Fig. 4 ), respectively, all affect RLP30/SCP Ss complex formation and, likely, are responsible for the non-functionality of these mutated receptors. RLP30 detects SCPs from fungi and oomycetes Homologs of SCP Ss exist in many fungi and oomycetes [12] . They typically contain a predicted signal peptide, seven conserved motifs (R1 to R7) and eight conserved cysteine residues (Supplementary Fig. 5a ), however, the absence of previously characterized protein domains hampers the prediction of their specific biological functions. Some SCPs have been reported to function as virulence factors with diverse modes of action [20] . However, deletion of the SCP Ss - homolog in B. cinerea ( SCP Bc /Bcplp1 ) or its homolog VmE02 in V. mali did not alter pathogenicity on various plants [12] , [21] (Supplementary Fig. 5b, c ), suggesting that these proteins either do not contribute significantly to virulence or act redundantly with others during infection. To assess whether SCP Ss homologs from other fungi and oomycetes display RLP30-dependent PAMP activity, homologs from B. cinerea (SCP Bc ) and Phytophthora infestans (SCP Pi ) were produced in P. pastoris (Supplementary Fig. 1e ). Similar to SCP Ss , SCP Bc and SCP Pi induced the production of ethylene and MAPK activation in wild-type or rlp30-2 /RLP30-YFP plants, but not in rlp30-2, sobir1-12 or bak1–5 bkk1–1 mutants or SCP Ss - insensitive accessions (Fig. 2a and Supplementary Fig. 5d, e ). Together, these data demonstrate that SCP Ss homologs, common among fungi and oomycetes, are perceived by the RLP30/SOBIR1/BAK1 receptor complex in Arabidopsis . Fig. 2: SCPs are sensed by RE02 and RLP30. a Ethylene accumulation in Arabidopsis wild-type plants (Col-0) or indicated mutants 4 h after treatment with water (mock), 1 μM nlp20, 1 µM SCP Ss , or homologs from B. cinerea ( Bc ) and Phytophthora infestans ( Pi ). b N. benthamiana plants were silenced for RE02 , and transiently transformed with RLP23-GFP , RLP30-GFP , or RE02-GFP , respectively. The TRV2:GUS construct was used as a control. Ethylene production was measured 4 h after treatment with water (mock), 1 μM nlp20, or 1 µM SCP Ss . c Ethylene accumulation in Arabidopsis rlp30-2 mutants or lines stably expressing RLP30-YFP or RE02-GFP (line 4 and 5) 4 h after treatment with water (mock), 1 μM nlp20, or 1 µM SCP Ss . Data points are indicated as dots ( n = 6) and plotted as box plots (center line, median; bounds of box, the first and third quartiles; whiskers, 1.5 times the interquartile range; error bar, minima and maxima). Statistically significant differences from control treatments are indicated (two-sided Student’s t test, *** P ≤ 0.001). Source data are provided as a Source data file. Each experiment was repeated three times with similar results. Full size image SCP Ss is sensed by RE02 in N. benthamiana SCP Ss recognition systems are present in both Brassicaceae and Solanaceae (Fig. 1d ), yet, reciprocal sequence similarity searches suggest absence of RLP30 from Solanaceae. The N. benthamiana receptor-like protein RE02 (RESPONSE TO VmE02) was recently identified to mediate the perception of VmE02, a cysteine-rich PAMP derived from V. mali with 55% identity to SCP Ss [12] , [22] . To compare the ligand specificity of RE02 with RLP30, RE02 expression in N. benthamiana was targeted by virus-induced gene silencing (VIGS), resulting in almost complete loss of SCP Ss -induced ethylene production (Fig. 2b and Supplementary Fig. 6a ). In contrast, leaves of silenced plants, either transiently transformed with RE02 -GFP or RLP30 -GFP exhibited clear SCP Ss sensitivity (Fig. 2b and Supplementary Fig. 6b ). Likewise, stable expression of RE02 –GFP also reconstituted responsiveness to SCP Ss in Arabidopsis rlp30-2 mutants (Fig. 2c and Supplementary Fig. 6c ). Hence, SCP Ss recognition is mediated by RE02 in N. benthamiana . RLP30 and RE02 evolved independently for at least 140 million years RLP30 and RE02 recognize the same microbial pattern but share only about 24% sequence identity (Supplementary Fig. 4b ). To investigate RLP30 and RE02 evolution, we analyzed the phylogenetic distribution of receptor proteins related to RLP30. We calculated a detailed phylogeny based on a dataset comprising A. thaliana protein sequences, those of other Brassicaceae, Fabaceae, Solanaceae, grape vine ( Vitis vinifera , member of the sister lineage to rosids and asterids), and Amborella trichopoda (the sister species to all other angiosperms) (Supplementary Fig. 7 ). Our data strongly support a sister group relationship of the RE02-like subfamily and the RLP30 subfamily with both subfamilies including members from Amborella . This indicates a split of the RLP30 and RE02 subfamilies in the lineage leading to all flowering plants, allowing these subfamilies to evolve independently for least 140 million years [23] . Hence, SCP sensor systems arose independently from convergent evolution. Interestingly, the RE02-like subfamily does not include any malvid protein sequences, suggesting that malvids lost RE02 -like genes, while in contrast RE02-like genes were copied multiple times in grape vine (Supplementary Fig. 7 ). Thus, we speculate that, compared to Solanaceae, immunity against microbial pathogens in malvids, including Brassicaceae or Fabaceae, might rely more strongly on RLP30 -related genes. Unlike the RE02-like subfamily, members of the RLP30-like subfamily were retained in all species analyzed and show lineage-specific expansions, as predicted previously by pre-computed phylogenetic trees from PhyloGene [24] . Within the Brassicaceae, 30 RLP30 -like genes are encoded by the A. thaliana genome. They form a monophyletic clade with other Brassicaceae genes supported by maximum bootstrap support, suggesting that they originate from a single gene copy in the lineage leading to Brassicaceae. Distinct perception of SCPs in Brassicaceae and Solanaceae Immunogenic activity of SCP Ss is sensitive to treatment with DTT (Supplementary Fig. 8a ), suggesting that perception by the RLPs RLP30 and RE02 depends on the tertiary structure of SCP Ss . The SCP Ss protein is predicted to form four disulfide bonds, most likely connecting cysteine residues C1 and C4, C2 and C3, C5 and C8 and C6 and C7, respectively (Fig. 3a ). Replacing individual cysteine residues in SCP Ss with serine leads to loss of activity and RLP30 complex formation in Arabidopsis for all eight substitutions (Fig. 3b and Supplementary Fig. 8b, c ). When testing the individual Cys substitutions for ethylene-inducing activity in N. benthamiana or tomato, we observed that only the four N-terminal Cys residues, forming the bonds C1-C4 and C2-C3, were required for ethylene-induction, while replacement of the other four Cys residues did not affect the activity (Fig. 3b and Supplementary Fig. 8d ). Hence, whereas RLP30 only senses intact SCP Ss , RE02-mediated perception requires only part of the SCP Ss tertiary structure. Fig. 3: SCP Ss sensing differs in Brassicaceae and Solanaceae. a Schematic representation of SCP Ss and derived truncations C1C5, C3C8, C1C4 and C3C5. Cysteine (C) residues are numbered and indicated as red lines, predicted disulfide bridges (DB, http://clavius.bc.edu/~clotelab/DiANNA/ ) are shown on top. SP, signal peptide. b , c Ethylene accumulation in A. thaliana Col-0, N. benthamiana or B. napus wild-type plants after 4 h treatment with water (mock), 1 µM SCP Ss , and SCP Ss with individual cysteine to serine mutations (C1S to C8S, according to cysteine numbering shown in a ) ( b ) or SCP Ss truncations depicted in a ( c ). Data points are indicated as dots ( n = 6) and plotted as box plots (center line, median; bounds of box, the first and third quartiles; whiskers, 1.5 times the interquartile range; error bar, minima and maxima). Statistically significant differences from mock treatments in the respective plants are indicated (two-sided Student’s t test, *** P ≤ 0.001). d Determination of EC 50 values of SCP Ss and the various SCP Ss truncations using ethylene accumulation in A. thaliana , N. benthamiana , or B. napus plants after treatment with increasing concentrations of recombinant SCP Ss versions (produced in Pichia ) or synthetic C3C5 (n.d, activity not detectable). Source data are provided as a Source data file. Each experiment was repeated three times with similar results. Full size image Consistent with the results of the individual cysteine replacements, a truncated form of SCP Ss , comprising C1 to C5 (C1C5), was active in tomato and N. benthamiana but not in Arabidopsis (Fig. 3c, d and Supplementary Fig. 8e ). C1C4, a variant of the protein further truncated from both the N- and the C-terminus but still comprising the first four Cys residues, proved inactive in Arabidopsis but also in N. benthamiana and tomato (Fig. 3c, d and Supplementary Fig. 8e ), indicating that in addition to the disulfide bonds also amino acids flanking the C1C4 peptide are important for immunogenic activity in solanaceous plants. Thus, SCP Ss is one of the very few identified ligands whose tertiary structure is important for PAMP activity similar to IF1-recognition by RLP32 [14] . Intriguingly, all SCP Ss mutants exhibited elicitor activity comparable to the wild-type SCP Ss in B. napus, B. rapa , and B. oleracea (Fig. 3b–d and Supplementary Fig. 8d, e ), indicating that in these Brassicaceae species SCP Ss -immunogenic activity is independent of cysteine-bridges and, thus, of its tertiary structure. Hence, at least two distinct SCP Ss -perception systems are present in Brassicaceae, one responding to intact SCP Ss protein (as in Arabidopsis ), and the other one responding to a SCP Ss -derived peptide (as in Brassica ssp.). As both C1C5 and C3C8 displayed activity in Brassicaceae, we generated the 36-amino-acid peptide C3C5 spanning the overlapping region of C1C5 and C3C8 (Fig. 3a ). C3C5, which contains only one cysteine residue (C4) and thus cannot form any disulfide bridge, was found to be nearly as active as intact SCP Ss in B. napus, B. rapa , and B. oleracea (Fig. 3c, d and Supplementary Fig. 8e ), indicating that this SCP Ss -fragment is sufficient to trigger immune responses in Brassica species. We therefore demonstrate that unlike RLP30-mediated recognition of intact SCP Ss in Arabidopsis , Brassica species can sense a small SCP Ss epitope that is distinct from the disulfide-bond containing peptide perceived in Solanaceae. In general, such large differences of sensor systems rather occur in distantly related plant families. However, similar to SCP Ss , PG perception also differs within the Brassicaceae family and A. thaliana , A. arenosa , and B. rapa perceive immunogenic PG fragments pg9(At), pg20(Aa) and pg36(Bra), respectively [15] . Thus, the perception diversity for SCP Ss or PG in closely related species within the same plant family could indicate adaptive processes in plant pathogen co-evolution in Brassicaceae. RLP30 senses Pseudomonas -derived PAMPs Intriguingly, rlp30 mutants have been found to be more susceptible to bacterial infection with P. syringae pv. phaseolicola ( Psp 1448A) [25] . We thus wondered whether RLP30 might also recognize a PAMP from Pseudomonads, despite the apparent absence of SCP Ss homologs in bacteria [12] . Using the chromatographic enrichment protocol established for SCFE1 [18] , we could detect elicitor-activity in culture media of different Pseudomonas species, such as Psp 1448A, Pst DC3000, P. fluorescens , P. protegens , and P. stutzeri (Fig. 4a ). Focusing on the activity from Psp , termed SCP-like Psp , we observed typical immune responses such as ethylene production, MAPK activation, as well as priming for resistance towards Pst DC3000 infection in Arabidopsis Col-0 wild-type plants and the rlp30-2 mutant complemented with RLP30 (Fig. 4b and Supplementary Fig. 9a ). SCP-like Psp also induced ethylene biosynthesis in fls2 efr and rlp32-2 mutants, indicating that activity was not due to the well-established bacterial PAMPs flagellin, EF-Tu or IF1 (Supplementary Fig. 9b ). In contrast, SCP-like Psp had no activity in the mutant rlp30- 2 , in nine of the SCP Ss -insensitive accessions, and in the sobir1-12 and bak1-5 bkk1-1 mutants (Fig. 4a and Supplementary Fig. 9c, d ), suggesting that perception of SCP-like Psp involves all the components required for perception of SCP Ss . So far, our attempts to determine the molecular identity of SCP-like Psp were not successful. However, much like SCP Ss , the immunogenic activity of SCP-like Psp was sensitive to treatment with DTT and proteases, but resistant to heat and SDS treatment, suggesting that it is likely also a protein stabilized by disulfide bridges (Supplementary Fig. 9e ). Fig. 4: Pseudomonads produce a RLP30-dependent elicitor activity. a Ethylene accumulation in Col-0 wild-type plants, rlp30-2 mutants or an rlp30-2 line complemented with a p35S::RLP30-YFP construct 4 h after treatment with water (mock), 1 μM SCP Ss or 1.5 μg/ml SCP-like from Pseudomonas syringae pv. tomato (Pst) , P. syringae pv. phaseolicola (Psp) , P. fluorescens (Pflu) , P. protegens (Ppr) , and P. stutzeri (Pstu) . b Bacterial growth in Col-0 wild-type plants, rlp30-2 mutants, or the rlp30-2/RLP30-YFP complementation line treated with water (mock), 1 μM nlp20, or 1.5 μg/ml SCP-like Psp 24 h before infiltration of Pst DC3000. Bacteria (colony forming units, CFU) were quantified in extracts of leaves 3 days after inoculation. c Ethylene accumulation in N. benthamiana ( Nb ) plants transiently expressing RLP23-GFP or RLP30-GFP and treated for 4 h with water (mock), 1 μM nlp20, or 1.5 μg/ml SCP-like Psp . Data points are indicated as dots ( n = 6 for a , c; n = 20 for b ) and plotted as box plots (center line, median; bounds of box, the first and third quartiles; whiskers, 1.5 times the interquartile range; error bar, minima and maxima). Statistically significant differences from Col-0 plants ( a ) or mock treatments ( b , c ) are indicated (two-sided Student’s t test, *** P ≤ 0.001). Source data are provided as a Source data file. Each experiment was repeated three times with similar results. Full size image RLP30 and RE02 differ in perception of SCP-like Psp SCP-like Psp showed activity in A. thaliana , B. rapa , and B. oleracea . Thus, species of the Brassicaceae family perceive SCPs and therefore have to encode functional RLP30 homologs (Supplementary Fig. 9f ). Interestingly, none of the species from the Solanaceae family tested showed responsiveness to bacterial SCP-like Psp (Supplementary Fig. 9f ). These species included N. benthamiana, S. pennellii, S. lycopersicum, S. tuberosum and C. annuum with functional SCP Ss perception, indicating that RE02 and solanaceous homologs do not respond to SCP-like Psp . Ectopic expression of RLP30 in N. benthamiana conferred sensitivity to SCP-like Psp , but not to nlp20 which required expression of RLP23 (Fig. 4c and Supplementary Fig. 9g ). Thus, RLP30, but not RE02, senses patterns from three microbial kingdoms. RLP30 expression in N. tabacum confers increased resistance to bacterial, fungal and oomycete pathogens Since RLP30 has the property of sensing PAMPs from microorganisms of three kingdoms, we introduced RLP30 into SCP Ss -insensitive N. tabacum plants. We observed that N. tabacum plants transiently expressing RLP30-GFP were responsive to SCP Ss and SCP-like Psp , albeit with only a moderate increase in production of ethylene (Supplementary Fig. 10a, b ). We wondered whether this might be due to a partial incompatibility of RLP30 with the endogenous tobacco SOBIR1. Indeed, co-expression of RLP30 with At SOBIR1 in N. tabacum established higher responses to SCP Ss and SCP-like Psp , whereas plants co-transformed with RLP30 and NbSOBIR1 or SlSOBIR1 showed responses as plants without additional SOBIR1 (Supplementary Fig. 10a, b ). Thus, we introduced RLP30-RFP together with the AtSOBIR1-GFP into N. tabacum and selected two stable transgenic lines ( #49 and #55 ) based on detectable expression of RLP30 and At SOBIR1 (Supplementary Fig. 10c ). Neither of the two transgenic lines exhibited autoimmune phenotypes as mock treatment did not induce ethylene accumulation and no elevated expression of salicylic acid marker gene PR-1a or jasmonic acid marker gene PDF1.2 could be detected in untreated plants (Fig. 5a and Supplementary Fig. 10a, d ). In contrast to wild-type tobacco plants, #49 and #55 transgenic lines clearly responded to SCPs or SCP-like Psp (Fig. 5a ). Importantly, when inoculated with the host-adapted, virulent bacterial pathogen P. syringae pv. tabaci , both transgenic lines exhibited less bacterial growth than wild-type plants (Fig. 5b ). Moreover, compared to wild-type plants, both transgenic lines also exhibited less symptom development upon infection with the necrotrophic fungus B. cinerea and the oomycete Phytophthora capsici (Fig. 5c, d ). Taken together, stable, ectopic expression of RLP30 in N. tabacum conferred sensitivity to SCPs and SCP-like Psp and rendered these transgenic plants more resistant to destructive bacterial, fungal, and oomycete pathogens. Fig. 5: RLP30 expression in N. tabacum confers increased resistance to bacterial, fungal, and oomycete pathogens. a Ethylene accumulation in N. tabacum wild-type plants (Wt) or two transgenic lines ( #49 and #55 ) stably expressing RLP30-RFP and AtSOBIR1-GFP after 4 h treatment with water (mock), 1 µM SCP from indicated sources, or 1.5 μg/ml SCP-like Psp . b Bacterial growth of P. syringae pv. tabaci in N. tabacum wild-type plants (Wt) or transgenic RLP30/SOBIR1 lines (#49 and #55). Bacteria (colony forming units, CFU) were quantified in extracts of leaves 3 days after inoculation. c B. cinerea infected area on leaves of N. tabacum wild-type plants (Wt) or transgenic RLP30/SOBIR1 lines (left, shown are representative leaves) and determination of lesion diameter on day 2 after drop inoculation (right). d Growth of Phytophthora capsici on leaves of N. tabacum wild-type plants (Wt) or transgenic RLP30/SOBIR1 lines by determination of lesion size (right) of lesions observed under UV light (left, shown are representative leaves) on day 2 after drop inoculation. Data points are indicated as dots ( n = 6 for a ; n = 20 for b , n = 10 for c , d ) and plotted as box plots (center line, median; bounds of box, the first and third quartiles; whiskers, 1.5 times the interquartile range; error bar, minima and maxima). Statistically significant differences from wild-type (Wt) plants are indicated (two-sided Student’s t test, *** P ≤ 0.001). Source data are provided as a Source data file. Each experiment was repeated three times with similar results. Full size image Plants harbor a tremendous number of potential receptor genes, however, their characterization is strictly dependent on knowledge of respective ligands. We identified here the ligand of the previously described RLP30 [18] as a secreted, small cysteine-rich protein (SCP). SCP Ss is widely distributed across fungi and oomycetes [12] and its tertiary structure is important for PAMP activity, features that are rare and as combination unprecedented among known PAMPs. Additionally, SCP perception also shows unique characteristics. Supplementary Fig. 11 summarizes our findings showing that SCP Ss and related elicitors do not only serve as ligands for RLP30 in Arabidopsis , but also for RE02 in N. benthamiana and a yet unknown Brassica PRR. RLP30 and RE02 share low similarity and all these PRRs moreover show distinct requirements for SCP Ss : RLP30 requires intact SCP Ss , Solanaceae receptors including RE02 sense the N-terminal part containing only two disulfide bonds and for SCP Ss perception in Brassica (except Arabidopsis ) a fragment of 36 amino acid is sufficient. Hence, the distinct perception mechanisms of the same fungal protein most likely arose through convergent evolution of LRR-RPs in different plant families. Convergent evolution of RLP30 and RE02 is supported by our phylogenetic analysis, indicating that RLP30 and RE02 subfamilies evolved independently for at least 140 million years. Moreover, RE02 and RLP30 have different protein structures with RE02 harboring 28 LRR motifs versus 21 LRRs in RLP30 and both proteins have highly divergent island domains. Based on the motif features within the island domain, RE02 (Kx 5 Y motif) and RLP30 (Hx 8 KG motif) are classified into two different clades [26] . Notably, the island domain of plant LRR-proteins was shown to participate in ligand binding [15] , [27] , explaining the different structural requirements of RLP30 and RE02 for SCP Ss perception and the ability of RLP30 to recognize a bacterial SCP-like pattern. Intriguingly, despite the broad capacity of multiple Brassicaceae and Solanaceae species to detect SCP Ss , multiple Arabidopsis ecotypes carry altered RLP30 receptors that do not recognize SCP Ss . Although RLP30 is considered a conserved LRR-RP and RLP30 sequences are present in most Arabidopsis ecotypes [28] , slight sequence variations might lead to functional diversification. Alternatively, accession-specific loss of RLP30 function might be explained by redundancy of Arabidopsis cell-surface immune receptors for fungal patterns such as SCPs, NLPs, PGs, oligogalacturonides or chitin perceived by Arabidopsis receptors RLP30, RLP23, RLP42, WAK1 or LYK5/CERK1, respectively [19] , [29] , [30] , [31] . This complexity is also reminiscent of Arabidopsis sensors for Pseudomonas -derived patterns [4] . SCP Ss -like sequences are not found in bacteria [12] , yet RLP30, but not RE02, confers recognition of SCP-like Psp from both pathogenic and beneficial Pseudomonas species. Hence, RLP30 is a unique receptor that can recognize most likely distinct ligands from fungi/oomycetes and bacteria. Such a broad detection range predestines PRRs such as RLP30 as a valuable genetic tool to boost crop immunity, and RLP30 expression in N. tabacum does indeed confer quantitative resistance to bacterial, fungal, and oomycete infections. Notably, RE02 also functions in Arabidopsis , indicating that the complex partner proteins are sufficiently conserved across wide taxonomic space, which is also supported by multiple reports on successful transfer of PRRs across taxa [14] , [19] , [32] , [33] . As RLP30, however, only modestly functions in tobacco without co-expressing AtSOBIR1, we propose that co-expression of heterologous PRR/co-receptor pairs may be deployed to overcome putative incompatibilities of ectopically expressed PRRs. Consequently, this way enhanced broad-spectrum resistance may be engineered as compared to expressing single PRRs alone. Plant materials and growth conditions Arabidopsis thaliana natural accessions [34] , [35] and mutant plants were grown in soil for 7-8 weeks in a growth chamber under short-day conditions (8 h photoperiod, 22 °C, 40–60% humidity). 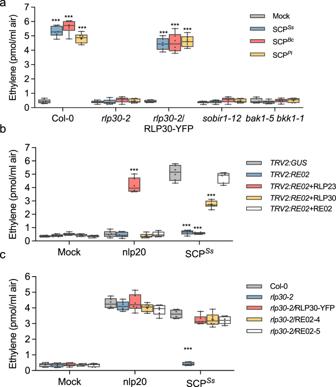Fig. 2: SCPs are sensed by RE02 and RLP30. aEthylene accumulation inArabidopsiswild-type plants (Col-0) or indicated mutants 4 h after treatment with water (mock), 1 μM nlp20, 1 µM SCPSs, or homologs fromB. cinerea(Bc) andPhytophthora infestans(Pi).bN. benthamianaplants were silenced forRE02, and transiently transformed withRLP23-GFP,RLP30-GFP, orRE02-GFP, respectively. TheTRV2:GUSconstruct was used as a control. Ethylene production was measured 4 h after treatment with water (mock), 1 μM nlp20, or 1 µM SCPSs.cEthylene accumulation inArabidopsis rlp30-2mutants or lines stably expressing RLP30-YFP or RE02-GFP (line 4 and 5) 4 h after treatment with water (mock), 1 μM nlp20, or 1 µM SCPSs. Data points are indicated as dots (n= 6) and plotted as box plots (center line, median; bounds of box, the first and third quartiles; whiskers, 1.5 times the interquartile range; error bar, minima and maxima). Statistically significant differences from control treatments are indicated (two-sided Student’sttest, ***P≤ 0.001). Source data are provided as a Source data file. Each experiment was repeated three times with similar results. Mutant lines and derived complemented transgenic lines are listed in Supplementary Table 2 . Solanaceae and Brassica plants were grown in a greenhouse at 23 °C under long-day conditions of 16 h of light and 60–70% humidity. Peptides Synthetic peptides flg22, nlp20, and SCP Ss C3C5 (SAYTCAAPAKSHLTAESDYWVFYWGNEGVSPGVGST) (GenScript) were prepared as 10 mM stock solutions in 100% dimethyl sulfoxide (DMSO) and diluted in water to the desired concentration before use. SCP Ss identification Partially purified SCFE1 fractions from S. sclerotiorum strain 1946 were used [18] . The most active fractions from eight rounds of fungal culture and the two-step cation-exchange chromatography purification protocol were pooled and dialyzed overnight in 2 l 25 mM MES, pH 7.0, at 4 °C in a dialysis membrane (ZelluTrans, nominal MWCO: 3.5; 46 mm, Roth), afterwards vacuum-filtrated through a cellulose acetate membrane (Ciro Manufacturing Corporation, pore size: 0.2μm) and loaded with a flow rate of 1 ml/min onto a Source 15S 4.6/100PE column (GE Healthcare) equilibrated with buffer A (50 mM MES, pH 5.4). After washing with buffer A, bound proteins were eluted with a linear gradient of buffer B (500 mM KCl, 50 mM MES, pH 5.4; 0–50% in 15 column volumes) and 500 μl fractions were collected using automated fractionation. LC-MS/MS sample preparation Three elicitor-active (B11 to B13, Supplementary Fig. 1b ), and two inactive (B9 and B15) fractions of SCFE1 (in 50 mM MES buffer pH 7.0 with varying concentration of KCl, depending on the elution time point) were selected for proteomics analysis. For each fraction a sample volume of 88 µl was used, which corresponded to a total protein content per fraction from 3.9 µg (B9) to 16.0 µg (B13), as determined using the BCA protein assay kit (Thermo Fisher Scientific). All samples were reduced (10 mM DTT, 30 min, 30 °C) and carbamidomethylated (55 mM CAA, 30 min, room temperature). Digestion of proteins was carried out by addition of trypsin (proteomics grade, Roche) at a 1/50 enzyme/protein ratio (w/w) and incubation at 37 °C overnight. Digests were acidified by addition of 0.5% (v/v) formic acid, and desalted using self-packed StageTips (three disks per micro-column, ø 1.5 mm, C18 material, 3 M Empore). The peptide eluates were dried to completeness and stored at −80 °C. For LC-MS/MS analysis all samples were resuspended in 11 µl 0.1% formic acid in HPLC grade water and 5 µl sample per measurement was injected into the mass spectrometer. LC-MS/MS data acquisition LC-MS/MS measurements were performed on a nanoLC Ultra1D+ (Eksigent, Dublin, CA) coupled online to a Q-Exactive HF-X mass spectrometer (Thermo Fisher Scientific). Peptides were loaded onto a trap column (ReproSil-pur C18-AQ, 5 µm, Dr. Maisch, 20 mm × 75 μm, self-packed) at a flow rate of 5 μl/min in 100% solvent A (0.1% formic acid in HPLC grade water). Subsequently, peptides were transferred to an analytical column (ReproSil Gold C18-AQ, 3 μm, Dr. Maisch, 400 mm × 75 μm, self-packed) and separated using a 50 min linear gradient from 4% to 32% of solvent B (0.1% formic acid in acetonitrile and 5% (v/v) DMSO) at 300 nl/min flow rate. Both nanoLC solvents contained 5% (v/v) DMSO to boost the nanoESI response of peptides. The eluate from the analytical column was sprayed via a stainless-steel emitter (Thermo Fisher Scientific) at a source voltage of 2.2 kV into the mass spectrometer. The transfer capillary was heated to 275 °C. The Q-Exactive HF-X was operated in data-dependent acquisition (DDA) mode, automatically switching between MS1 and MS2 spectrum acquisition. MS1 spectra were acquired over a mass-to-charge ( m/z ) range of m / z 350–1400 at a resolution of 60,000 using a maximum injection time of 45 ms and an AGC target value of 3e6. Up to 18 peptide precursors were isolated (isolation window m / z 1.3, maximum injection time 25 ms, AGC value 1e5), fragmented by high-energy collision-induced dissociation (HCD) using 26% normalized collision energy and analyzed at a resolution of 15,000 with a scan range from m / z 200–2000. Precursor ions that were singly charged, unassigned, or with charge states >6+ were excluded. The dynamic exclusion duration of fragmented precursor ions was 25 s. LC-MS/MS data analysis Peptide identification and quantification was performed using MaxQuant (version 1.5.3.30) [36] . MS2 spectra were searched against a Sclerotinia sclerotiorum protein database (assembly accession number PRJNA348385 , 11130 protein sequence entries), supplemented with common contaminants (built-in option in MaxQuant). Carbamidomethylated cysteine was set as fixed modification and oxidation of methionine and N-terminal protein acetylation as variable modifications. Trypsin/P was specified as proteolytic enzyme. Precursor tolerance was set to 4.5 ppm, and fragment ion tolerance to 20 ppm. Results were adjusted to 1% false discovery rate (FDR) on peptide spectrum match (PSM) and protein level employing a target-decoy approach using reversed protein sequences. The minimal peptide length was defined as 7 amino acids, the “match-between-run” function was enabled (default settings). To assess and quantitatively compare the concentrations of the detected proteins the “intensity based absolute quantification” (iBAQ) [37] algorithm was employed. The detected 22 proteins were further filtered and prioritized according to the following characteristics: (1) good correlation between the elicitor activity profile and the measured mass spectrometric protein intensity over the five investigated SCFE1 fractions; (2) presence of a predicted signal peptide sequence (using the SignalP v.6.0 server) [38] ; (3) protein molecular weight in the range between 10 to 30 kDa; (4) high cysteine content relative to protein length; (5) detection of at least two unique peptides per protein (Supplementary Table 1 ). SCP Ss expression and purification For expression of SCP Ss in N. benthamiana leaves, the SCP Ss sequence was cloned into the pBIN-plus vector with a C-terminal GFP tag [15] . Agrobacterium tumefaciens strain GV3101 carrying pBIN-plus-SCP Ss was infiltrated into leaves of 4–6-week-old N. benthamiana plants. At 48 h post agro-infiltration, leaves were vacuum-infiltrated with 0.5 M NaCl, 0.4 M Na 2 HPO 4 and 0.4 M NaH 2 PO 4 and the apoplastic wash-fluid containing SCP Ss (SCP Ss -AWF) was collected by centrifugation at 1500 × g for 20 min and 4 °C. For recombinant protein expression in Pichia pastoris KM71H (Multi-Copy Pichia Expression Kit Instructions, Thermo Fisher Scientific), constructs encoding SCP Ss , SCP Bc , SCP Pi , truncated SCP Ss versions and cysteine-to-serine replacements (all without signal peptide and Stop codon) were cloned into the secretory expression plasmid pPICZalphaA (Thermo Fisher Scientific). Individual cysteine to serine replacements in SCP Ss were amplified from synthetic genes (gBlocks, Integrated DNA Technologies) using primers extended by restriction sites Eco Rl and Bam HI and cloned into pPICZalphaA. Sequence information on primers and synthetic genes used in this study can be found in Supplementary Tables 3 and 5 . Protein purification from P. pastoris culture medium was achieved by affinity chromatography on 5 ml HisTrapFF column (GE Healthcare; equilibrated in 20 mM Tris-HCl, 200 mM NaCl, pH 8.0), following washing (20 mM Tris-HCl, 200 mM NaCl, 20 mM imidazole, pH 8.0) and elution (buffer gradient 0–500 mM imidazole in equilibration buffer). Recombinant protein expression was verified by concentration determination using the Bradford method and by Western Blot analysis using the anti-His antibody (dilution 1:1000, Abcam). SCP-like purification from Pseudomonas ssp Pseudomonas strains ( Pseudomonas syringae pv . tomato DC3000, Pseudomonas syringae pv . phaseolicola 1448A, Pseudomonas protegens Pf-5, Pseudomonas fluorescens SBW25, Pseudomonas stutzeri DSM10701) were grown in baffled flasks (200 ml medium in 1 l flask) in liquid PDB medium (24 g/l Potato Dextrose Broth, Duchefa) for 12 h at 21 °C with 210 rpm shaking. The culture medium was centrifuged at 6000 rpm for 20 min and then vacuum-filtrated through a filter paper (MN 615, Macherey-Nagel) and subjected to a two-step cation exchange chromatography protocol using an ÄKTA Explorer FPLC system (GE Healthcare) kept at 4 °C. In a first step, the culture filtrate was loaded onto HiTrap SP FF column(s) (GE Healthcare) equilibrated in buffer A (50 mM MES, pH 5.4) at a flow rate of up to 15 ml/min. After washing with buffer A, a 100% elution step with buffer B (500 mM KCl, 50 mM MES, pH 5.4) was performed at a flow rate of 1–2 ml/min and the elution peak was monitored with OD280nm, OD254nm and OD214nm and collected manually. The collected eluate was dialyzed against 2 l 25 mM MES, pH 5.4, overnight at 4 °C in a dialysis membrane (ZelluTrans, nominal MWCO: 3.5; 46 mm, Roth), afterwards vacuum-filtrated through a cellulose acetate membrane (Ciro Manufacturing Corporation, pore size: 0.2 μm) and loaded with a flow rate of 1 ml/min onto a Source 15 S 4.6/100PE column (GE Healthcare) equilibrated with buffer A. After washing with buffer A the bound proteins were eluted with a linear gradient of buffer B (0–50% in 10 column volumes) and 500 μl fractions were collected using automated fractionation. 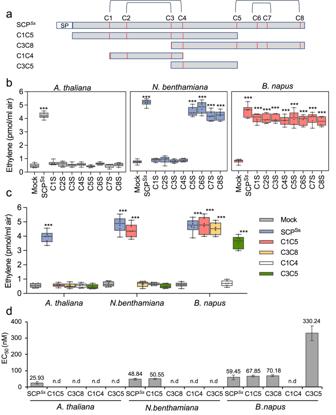Fig. 3: SCPSssensing differs in Brassicaceae and Solanaceae. aSchematic representation of SCPSsand derived truncations C1C5, C3C8, C1C4 and C3C5. Cysteine (C) residues are numbered and indicated as red lines, predicted disulfide bridges (DB,http://clavius.bc.edu/~clotelab/DiANNA/) are shown on top. SP, signal peptide.b,cEthylene accumulation inA. thalianaCol-0,N. benthamianaorB. napuswild-type plants after 4 h treatment with water (mock), 1 µM SCPSs, and SCPSswith individual cysteine to serine mutations (C1S to C8S, according to cysteine numbering shown ina) (b) or SCPSstruncations depicted ina(c). Data points are indicated as dots (n= 6) and plotted as box plots (center line, median; bounds of box, the first and third quartiles; whiskers, 1.5 times the interquartile range; error bar, minima and maxima). Statistically significant differences from mock treatments in the respective plants are indicated (two-sided Student’sttest, ***P≤ 0.001).dDetermination of EC50values of SCPSsand the various SCPSstruncations using ethylene accumulation inA. thaliana,N. benthamiana, orB. napusplants after treatment with increasing concentrations of recombinant SCPSsversions (produced inPichia) or synthetic C3C5 (n.d, activity not detectable). Source data are provided as a Source data file. Each experiment was repeated three times with similar results. Generation of transgenic plants For the generation of transgenic rlp30-2 lines expressing p35S::RE02-GFP , the coding sequence of RE02 extended by Bsa I cleavage sites (Supplementary Table 3 ) was cloned into the pGEM®-T vector (Promega). The cauliflower mosaic virus 35 S promoter, RE02 coding sequence and GFP-tag were assembled via golden gate cloning in the vector LII_F_1-2_-_BB10c [39] and constructs were transformed into rlp30-2 by floral dipping. For 35S-promoter-driven stable expression of RLP30-YFP in rlp30-2 mutants or RLP30-RFP and SOBIR1-GFP in N. tabacum L . var. Samsun NN, RLP30 and SOBIR1 coding sequences were first cloned into pCR™8/GW/TOPO™ (Thermo Fisher Scientific) and subsequently fused via Gateway cloning to a C-terminal YFP (pB7YWG2 [40] ), RFP (pB7RWG2 [40] ) or GFP (pK7FWG2 [40] ), respectively. Primers used are listed in Supplementary Table 3 . For stable transformation, A. tumefaciens GV3101 carrying the desired constructs were grown in LB medium with appropriate antibiotics. For Arabidopsis transformation, bacterial cells were harvested and resuspended in 5% (w/v) Sucrose, 0.02% (v/v) Silwet at an O.D. of 0.8 and buds of 6–8-week-old rlp30-2 mutants were dipped for approximately 1.5 min. The T1 generation was selected on 0.2% (v/v) BASTA. For Nicotiana tabacum transformation, cells were resuspended in 10 mM MgCl 2 . Leaf pieces were incubated in the bacterial suspension for 3 min, subsequently transferred to MS medium with 2% sucrose, and incubated for 48 h in the dark. Transgenic calli were selected on MS medium with corresponding antibiotics. Transgenic plants selected in sterile culture were transferred to soil and grown in the greenhouse under long day conditions. Protein expression in transgenic lines was verified by immunoblotting using anti-RFP (Abcam) and anti-GFP (Thermo Fisher Scientific) antibodies and response to SCFE1 [18] . Transient protein expression and co-immunoprecipitations For 35S-promoter-driven transient protein expression in N. benthamiana or N. tabacum [19] , coding sequences of respective genes were amplified using the primers listed in Supplementary Table 3 , cloned into pCR™8/GW/TOPO™ (Thermo Fisher Scientific) and subsequently recombined via Gateway cloning into pGWB5 (C-terminal GFP-tag), pGWB14 (C-terminal HA-tag), or pGWB17 (C-terminal Myc-tag) [41] . Likewise, a pENTR/D-Topo (Thermo Fisher Scientific) clone containing the coding sequence for NbSOBIR1 [42] was recombined with pGWB14, p35S::SlSOBIR1-HA in pGWB14 and constructs for AtSOBIR1-HA , BAK1-myc and RLP23-GFP have been described previously [19] , [43] . For SCP Ss -binding assays, native SCP Ss -Myc (pGWB17) or Cys-to-Ser replacement mutants (Supplementary Table 5 ) together with RLP30-GFP (pGWB5) from different Arabidopsis accessions was transiently co-expressed in N. benthamiana . 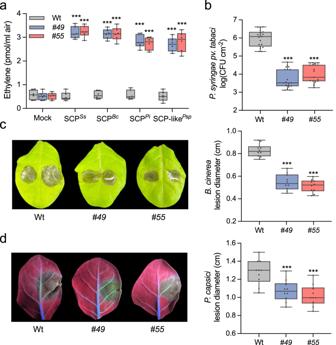Fig. 5: RLP30 expression inN. tabacumconfers increased resistance to bacterial, fungal, and oomycete pathogens. aEthylene accumulation inN. tabacumwild-type plants (Wt) or two transgenic lines (#49and#55) stably expressing RLP30-RFP and AtSOBIR1-GFP after 4 h treatment with water (mock), 1 µM SCP from indicated sources, or 1.5 μg/ml SCP-likePsp.bBacterial growth ofP. syringaepv.tabaciinN. tabacumwild-type plants (Wt) or transgenicRLP30/SOBIR1lines (#49 and #55). Bacteria (colony forming units, CFU) were quantified in extracts of leaves 3 days after inoculation.cB. cinereainfected area on leaves ofN. tabacumwild-type plants (Wt) or transgenicRLP30/SOBIR1lines (left, shown are representative leaves) and determination of lesion diameter on day 2 after drop inoculation (right).dGrowth ofPhytophthora capsicion leaves ofN. tabacumwild-type plants (Wt) or transgenicRLP30/SOBIR1lines by determination of lesion size (right) of lesions observed under UV light (left, shown are representative leaves) on day 2 after drop inoculation. Data points are indicated as dots (n= 6 fora;n= 20 forb,n= 10 forc,d) and plotted as box plots (center line, median; bounds of box, the first and third quartiles; whiskers, 1.5 times the interquartile range; error bar, minima and maxima). Statistically significant differences from wild-type (Wt) plants are indicated (two-sided Student’sttest, ***P≤ 0.001). Source data are provided as a Source data file. Each experiment was repeated three times with similar results. On day 2, leaf material was harvested and protein extracts were subjected to immunoprecipitation using GFP-Trap beads (ChromoTek). 200 mg ground leaf material was subjected to protein extraction and immunoprecipitation using GFP-Trap beads (ChromoTek) [19] . Proteins were detected by immunoblotting with tag-specific antibodies raised against epitope tags GFP (dilution 1:5000), HA (dilution 1:3000) or Myc (dilution 1:5000, all Thermo Fisher Scientific), followed by staining with secondary antibodies coupled to horseradish peroxidase and ECL (Cytiva). Plant immune responses Ethylene production was induced in three leaf pieces floating on 0.5 ml 20 mM MES buffer pH 5.7 and the indicated elicitors [44] . After incubation for 4 h, 1 ml air was drawn from sealed assay tubes and the ethylene content was measured by gas chromatography (GC-14A, Shimadzu). ROS accumulation was measured in one leaf piece per well placed in a 96-well plate (Greiner BioOne) containing 100 μl of a solution with 20 μM luminol derivative L-012 (Wako Pure Chemical Industries) and 20 ng/ml horseradish peroxidase (Applichem) [44] . Luminescence was measured in 2 min intervals both before (background) and for up to 60 min after PAMP or mock treatment using a Mithras LB 940 luminometer (Berthold Technologies). For MAPK activity assays, treated leaf material was harvested after indicated times and frozen in liquid nitrogen. Proteins were extracted with 20 mM Tris-HCl pH 7.5, 150 mM NaCl, 1 mM EDTA, 1% Triton X-100, 0.1% SDS, 5 mM DTT, Complete Protease Inhibitor Mini, EDTA-free (Roche), PhosStop Phosphatase Inhibitor Cocktail (Roche), separated via 10% SDS-PAGE, and transferred to nitrocellulose. 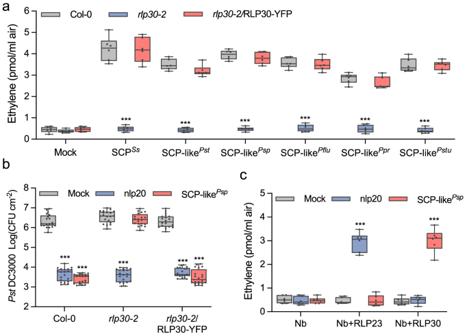Activated MAPKs were detected by protein blotting using the rabbit anti-phospho-p44/42-MAPK antibody (Cell Signalling Technology, 1:1000 dilution) [44] . Fig. 4: Pseudomonads produce a RLP30-dependent elicitor activity. aEthylene accumulation in Col-0 wild-type plants,rlp30-2mutants or anrlp30-2line complemented with ap35S::RLP30-YFPconstruct 4 h after treatment with water (mock), 1 μM SCPSsor 1.5 μg/ml SCP-like fromPseudomonas syringaepv.tomato (Pst),P. syringaepv.phaseolicola (Psp),P. fluorescens (Pflu),P. protegens (Ppr), andP. stutzeri (Pstu).bBacterial growth in Col-0 wild-type plants,rlp30-2mutants, or therlp30-2/RLP30-YFPcomplementation line treated with water (mock), 1 μM nlp20, or 1.5 μg/ml SCP-likePsp24 h before infiltration ofPstDC3000. Bacteria (colony forming units, CFU) were quantified in extracts of leaves 3 days after inoculation.cEthylene accumulation inN. benthamiana(Nb) plants transiently expressing RLP23-GFP or RLP30-GFP and treated for 4 h with water (mock), 1 μM nlp20, or 1.5 μg/ml SCP-likePsp. Data points are indicated as dots (n= 6 fora, c;n= 20 forb) and plotted as box plots (center line, median; bounds of box, the first and third quartiles; whiskers, 1.5 times the interquartile range; error bar, minima and maxima). Statistically significant differences from Col-0 plants (a) or mock treatments (b,c) are indicated (two-sided Student’sttest, ***P≤ 0.001). Source data are provided as a Source data file. Each experiment was repeated three times with similar results. RT-qPCR analysis in transgenic RLP30-RFP- and AtSOBIR1-GFP-expressing tobacco lines #49 and #55 was performed using gene specific primers for NtPR1 and NtPDF1.2 and NtACT9 as house-keeping gene as listed in Supplementary Table 4 . Plant infections Leaves of 6–8-week-old Arabidopsis plants were primed by leaf infiltration with 1 μM nlp20, 1 µM SCP Ss or SCP-like Psp , or water (mock treatment) and after 24 h inoculated with Pseudomonas syringae pv . tomato DC3000 ( Pst DC3000) by leaf infiltration with a final cell density of 10 4 colony-forming units (CFU) per ml 10 mM MgCl 2 . Bacterial populations were determined 3 d after infiltration [45] . N. tabacum plants were likewise infected with P. syringae pv . tabaci [46] at a final cell density of 10 5 CFU/ml and harvested after 4 days. For fungal infection, spores of B. cinerea isolate B05.10 or SCP Bc depletion mutant Δ SCP Bc /Bcplp1 [21] (lines 45 and 46) were diluted to a final concentration of 5 ×10 6 spores per ml in potato dextrose broth and 5-µl drops were used for leaf inoculation. Lesion sizes were determined after 2 d by determining the average lesion diameter. N. tabacum leaves inoculated with 0.8 cm fresh mycelial plugs of Phytophthora capsici grown on V8 juice agar were clipped and kept in the dark in plastic boxes to obtain high humidity. Lesion diameters were measured at 48 hpi using UV light. For Agrobacterium -mediated virus-induced gene silencing (VIGS) [42] , a 300 bp fragment of RE02 was amplified using primers listed in Supplementary Table 3 and cloned into vector pYL156 [47] ( TRV2::RE02 ), as control the TRV2::GUS construct was used [42] . Gene silencing was verified by measuring RE02 transcript levels versus NbActin transcript levels using quantitative RT-PCR [28] with primers listed in Supplementary Table 4 . Phylogeny reconstruction Full-length protein sequences, obtained from Ngou et al. [48] (a) and BLAST searches [49] on Phytozome [50] (b) or Uniprot [51] (c), of A. thaliana (a, b), B. rapa (a), M. truncatula (b), V.vinifera (b), S. lycopersicum (a, b), S. tuberosum (b), N. benthamiana (a), N. sylvestris (c) and A. trichopoda (b) were aligned using MAFFT [52] (--localpair --maxiterate 10000 --reorder). The phylogenetic tree was constructed using IQTree [53] (-T AUTO -m TEST -b 50 -con). Statistics and reproducibility No statistical methods were used to predetermine sample size. The experiments were not randomized. The investigators were not blinded to allocation during experiments and outcome assessment. Data were plotted using GraphPad Prism 9. Data were represented as the mean ± S.D. or as box-and-whisker plots in which the center line indicates the median, the bounds of the box indicate the 25th and 75th percentiles, and the whiskers indicate 1.5 times the interquartile range. Unless otherwise stated, graphs present data from a single experiment. No data were excluded from analyses. Data were analyzed with a two-sided Student’s t test using Microsoft Office Excel. A summary of statistical analyses is provided in Source data. Reporting summary Further information on research design is available in the Nature Portfolio Reporting Summary linked to this article.